Middle Eocene greenhouse warming facilitated by diminished weathering feedback 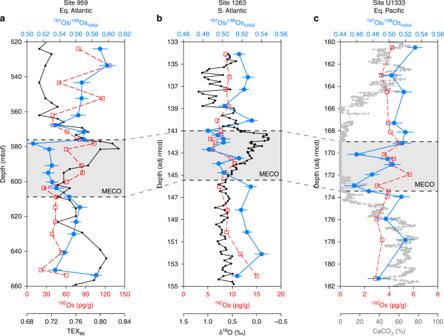Fig. 1 Osivalues (in blue) and192Os concentrations (in red) for the analyzed middle Eocene sediments from the three different sites.aODP Site 959;bODP Site 1263;cIODP Site U1333. The MECO interval is defined based on TEX86values for Site 959 (in black; Cramwinckel et al.13) and bulk carbonate stable oxygen isotope ratios (δ18O) for Site 1263 (in black; Bohaty et al.10). The MECO is characterized by low carbonate content at Site U1333 (in grey; Westerhold et al.84). The error bars indicate fully propagated analytical uncertainties (2σ) The Middle Eocene Climatic Optimum (MECO) represents a ~500-kyr period of global warming ~40 million years ago and is associated with a rise in atmospheric CO 2 concentrations, but the cause of this CO 2 rise remains enigmatic. Here we show, based on osmium isotope ratios ( 187 Os/ 188 Os) of marine sediments and published records of the carbonate compensation depth (CCD), that the continental silicate weathering response to the inferred CO 2 rise and warming was strongly diminished during the MECO—in contrast to expectations from the silicate weathering thermostat hypothesis. We surmise that global early and middle Eocene warmth gradually diminished the weatherability of continental rocks and hence the strength of the silicate weathering feedback, allowing for the prolonged accumulation of volcanic CO 2 in the oceans and atmosphere during the MECO. These results are supported by carbon cycle modeling simulations, which highlight the fundamental importance of a variable weathering feedback strength in climate and carbon cycle interactions in Earth’s history. The chemical weathering of silicate rocks represents a negative feedback mechanism that is generally considered to modulate atmospheric CO 2 levels and Earth’s climate on geological timescales [1] , [2] . This phenomenon has been studied for various carbon cycle perturbations and episodes of global warming in the geological past, including Pleistocene deglaciations, the Paleocene-Eocene Thermal Maximum (PETM; ~56 Ma), and the Cretaceous and Jurassic Oceanic Anoxic Events (OAEs), mainly through the application of isotope ratios of marine sediments that are sensitive to shifts in weathering fluxes or compositions on the appropriate timescales [3] , [4] , [5] . For many of these phases, it is now relatively well established that enhanced continental weathering contributed to CO 2 drawdown and climatic recovery [4] , [6] , [7] . However, the available data spanning the Middle Eocene Climatic Optimum (MECO; ~40 Ma) pose questions regarding the functioning of the weathering feedback [8] . Over a period of ~500 kyr, global ocean temperatures rose gradually by up to ~5 °C in association with an increase in atmospheric CO 2 concentrations, sourced from a reservoir with a stable carbon isotopic composition (δ 13 C) close to that of the ocean [9] , [10] , [11] , [12] , [13] . Importantly, the inferred rise in atmospheric CO 2 and temperature over ~500 kyr during the MECO should have led to increased weathering and alkalinity supply to the oceans, but reconstructions show that the oceans acidified [8] , [10] . Therefore, reconstructing the global weathering response during the MECO is instrumental to improving our fundamental understanding of carbon cycle dynamics on such intermediate timescales of ~500 kyr [8] . A promising proxy to reconstruct changes in continental weathering during the MECO is the osmium isotope ratio of marine sediments at the time of deposition ( 187 Os/ 188 Os initial , or Os i ) [14] , [15] . The 187 Os/ 188 Os ratio of the global ocean is governed by the relative input of radiogenic Os ( 187 Os/ 188 Os = ~1.4) through continental weathering of ancient crustal rocks, and the relative input of unradiogenic Os ( 187 Os/ 188 Os = 0.13) through hydrothermal activity at mid-ocean ridges and weathering of fresh mantle-derived rocks, with additional contributions from extraterrestrial sources [14] . Osmium is a quasi-conservative element that is well-mixed in the ocean, and has a short oceanic residence time (generally ~10 4 yr in the open ocean, but residence times of ~10 3 yr have been inferred for very restricted settings) [14] , [16] . Variations in the 187 Os/ 188 Os ratio of seawater are thus indicative of changes in continental weathering relative to the other sources on timescales shorter than, or similar to, climate and carbon cycle processes such as greenhouse warming, ocean acidification, and carbonate compensation [14] , [15] . Seawater Os is incorporated in the metalliferous and organic phases of marine sediments without isotopic fractionation, and remains a closed isotopic system from the time of deposition [17] , [18] , [19] . As such, Os i values are calculated on the basis that radiogenic 187 Os ingrowth is derived solely from post-depositional 187 Re (rhenium) decay. Shifts to higher (radiogenic) Os i values, which are attributed to a global increase in continental silicate weathering rates, have been recorded for carbon cycle perturbations such as the Toarcian OAE and the PETM and Eocene Thermal Maximum 2 (ETM2) transient global warming events [5] , [15] , [20] . A second parameter that is often used to constrain changes in continental weathering is the carbonate compensation depth (CCD). The CCD is the depth in the oceans at which carbonate delivery is balanced by carbonate dissolution, and is modulated by the interplay of volcanic CO 2 degassing, the weathering of silicate rocks and organic-rich sediments on land, and the burial of marine carbonates and organic carbon [21] . As such, changes in the position of the CCD as reflected in sediments play a crucial role in reconstructions of carbon cycle change, both on multi-million year timescales and during transient perturbations such as the MECO [22] . In this study, we present Os i records of marine sediments from three locations in different ocean basins in combination with a compilation of published CCD records [8] to reconstruct global changes in continental weathering during the MECO. Rather than an Os i increase expected from globally enhanced weathering, we document a modest global Os i decrease during the MECO that may represent an episode of enhanced volcanism and/or associated basalt weathering. In fact, prolonged CCD shoaling precludes an increase in total continental weathering rates in response to CO 2 rise and greenhouse warming. We employ a series of simulations with the carbon cycle model LOSCAR [23] together with an independent osmium cycle model to demonstrate that this combination of observations can only be successfully reconciled on MECO timescales by invoking enhanced volcanism together with a diminished continental weathering feedback. Finally, we surmise that such a reduced silicate weathering feedback may have resulted from a progressive decrease in the weatherability of the continents during the Eocene. A variable silicate weathering feedback strength may have been important for other enigmatic climate and carbon cycle perturbations in Earth’s history. Middle Eocene osmium isotope records We present Re-Os data and Os i values for middle Eocene sediments from Ocean Drilling Program (ODP) Site 959 in the equatorial Atlantic along the African continental margin, ODP Site 1263 on the Walvis Ridge in the South Atlantic, and Integrated Ocean Drilling Program (IODP) Site U1333 in the equatorial Pacific (Fig. 1 ; Supplementary Data 1 ; Supplementary Figs. 1 – 3 ). The Re and Os abundances are significantly enriched in the relatively organic-rich, siliceous sediments of Site 959 (Re = 10–60 ppb, Os = 100–300 ppt) relative to the carbonate-rich pelagic sediments of Sites 1263 and U1333 (Re = 0.02–0.2 ppb, Os = 10–40 ppt). The abundances of 192 Os, the Os isotope best representing the amount of hydrogenous Os chelated by organic matter at the time of deposition [24] , increase slightly over the study interval at Site 959, but are essentially stable at the other two sites (Fig. 1 ). We calculate Os i values of 0.46 to 0.60 at all study sites (Fig. 1 ), which is in good agreement with previously published middle Eocene Os i values from Site 959 sediments [25] , [26] and with Os i values from ferromanganese crusts that document a progressive increase in the 187 Os/ 188 Os composition of seawater during the Cenozoic [27] , [28] , [29] (Fig. 2 ). Fig. 1 Os i values (in blue) and 192 Os concentrations (in red) for the analyzed middle Eocene sediments from the three different sites. a ODP Site 959; b ODP Site 1263; c IODP Site U1333. The MECO interval is defined based on TEX 86 values for Site 959 (in black; Cramwinckel et al. [13] ) and bulk carbonate stable oxygen isotope ratios (δ 18 O) for Site 1263 (in black; Bohaty et al. [10] ). The MECO is characterized by low carbonate content at Site U1333 (in grey; Westerhold et al. [84] ). The error bars indicate fully propagated analytical uncertainties (2 σ ) Full size image Fig. 2 Comparison of Os i records from the MECO with Os i records from the PETM and ETM2, shown against the overall Os i evolution of the Cenozoic and the relative weathering feedback strength of the Cenozoic. a MECO data from Site 959 (in red), Site 1263 (in blue) and Site U1333 (in green) plotted against age (GTS2012) [74] . See Methods for discussion of the age models for the study sites. b MECO data from Sites 959, 1263, and U1333 (this study); PETM and ETM2 data from DSDP Site 549 (in purple) as published in Peucker-Ehrenbrink & Ravizza [15] ; Cenozoic data from ferromanganese crusts D11 and CD29 (in black) as published in Klemm et al. [27] and Burton [28] , respectively, based on the updated age model of Nielsen et al. [29] . c Model estimates of the relative continental weathering feedback strength of the Cenozoic as published in Caves et al. [57] , based on their CO 2 scenario 1 and a logarithmic expression for the weathering feedback Full size image At Site 959, the Os i values range between approximately 0.56 and 0.60 for most of the middle Eocene study interval, with the exception of a decrease to 0.51 during the MECO at ~580 mbsf (Fig. 1 ). Importantly, the lack of an increase in the Os i values during the MECO implies that weathering rates of felsic silicate rocks did not increase in response to CO 2 rise and accompanied warming, while such an increase would be expected from theory and published Os i records from analogous carbon cycle perturbations [3] , [7] , [15] (Fig. 2b ). Furthermore, the relative invariability of both the Os i records and the 192 Os abundances—which scale to organic matter content—implies that the balance of Os fluxes to the oceans and uptake of Os in sedimentary organic matter did not appreciably change during the MECO. Although the magnitude of the negative Os i shift at Site 959 is small (~0.05), it exceeds the maximum analytical uncertainty (2 σ = 0.01) by a factor of 5. The shift starts at the onset of MECO warming and is also present at Sites 1263 and U1333, where it is similar in magnitude (Figs. 1 , 2 ). Interestingly, the Os i profile of Site U1333 is characterized by two separate excursions to lower, less radiogenic values rather than the gradual and continuous decrease that is observed at Site 959. The Os i profile at Site 1263 shows trends intermediate to Sites 959 and U1333. Nevertheless, the lowest Os i values in all three records occur toward the end of the MECO, which is coincident with the peak warming phase [10] . In addition, the return towards pre-MECO values is synchronous with the termination of the MECO at all three sites, implying that the Os i shift lasted for the entire duration of the event (~500 kyr). The absolute Os i values differ slightly between sites, likely because of differences in coastal proximity and oceanographic setting [30] , [31] . However, the general timing and magnitude of the Os i shift are reproduced at all sites, indicating that the Os i shift records a change in the 187 Os/ 188 Os composition of the global ocean. The global character and synchroneity of the Os i shift at the end of the MECO also indicate that osmium isotope stratigraphy is a promising tool for correlation of the event between sites in future studies (Fig. 2a ). In principle, the modest negative Os i shift during the MECO may be caused by an increase in the unradiogenic Os flux from hydrothermal and/or extraterrestrial sources, a decrease in the radiogenic Os flux from continental weathering, or a decrease in the 187 Os/ 188 Os composition of the continental weathering flux through a transient change in the exposure of different rock types, such as basalts [7] . There is no evidence for an extraterrestrial impact during the MECO. Furthermore, a reduction in continental silicate weathering rates during an episode of greenhouse warming seems paradoxical and unlikely, even though our Os i records clearly show no evidence of the expected increase in continental weathering. It is difficult to exclude a warming-induced change in regional climates and precipitation patterns—which could have affected the contributions of rock types with different 187 Os/ 188 Os compositions to the continental weathering flux [3] , [32] —as a cause for the Os i shift. However, this would still require a different cause for MECO warming. Finally, the Os i shift could reflect a short-lived increase in mid-ocean ridge hydrothermal activity or an episode of increased volcanism and associated weathering of mafic silicate rocks [24] , [33] , [34] . Mass balance calculations with a progressive two-component mixing model that involves seawater and basalts (see Methods; Supplementary Data 2 ) show that the Os i shift across the MECO may correspond to a 10–15% increase in the contribution of the mantle-derived Os flux relative to the continental Os flux. Although there is no indication for the emplacement of a large igneous province during the middle Eocene [8] , an episode of volcanic activity at mid-ocean ridges or on land could have increased the Os flux from basalts, and consequently resulted in a decrease of the 187 Os/ 188 Os composition of the oceans that is consistent with our Os i records. Moreover, enhanced volcanism would provide a mechanism for the atmospheric CO 2 rise that has been inferred for the MECO [8] , [11] , perhaps similar to the Late Cretaceous episode of greenhouse warming associated with volcanic eruptions from the Deccan Traps [33] , [35] , [36] . Potential events that have been dated at approximately the right age in the middle Eocene include (1) a pulse of metamorphic decarbonation associated with Himalayan uplift and metamorphism [37] , [38] , (2) increased arc volcanism around the Pacific rim [39] and especially in the Caribbean, related to an ignimbrite flare-up in the Sierra Madre Occidental of Mexico [40] , [41] , [42] , (3) an episode of magmatism in the East African Rift zone [43] , in particular in Southern Ethiopia and Northern Kenya [44] , [45] , and/or (4) mid-ocean ridge volcanism in the North Atlantic, due to rifting in East Greenland and activity of the Iceland hotspot [46] , [47] , [48] . However, the timing and magnitude of these events are at present not sufficiently well resolved to establish a direct causal link with the MECO. Additionally, it is unclear if increased Himalayan uplift and metamorphism would be compatible with the observed negative Os i shift, as the Himalayas are generally considered to contribute relatively radiogenic Os to the continental weathering flux [49] , [50] . Yet, the effects of Himalayan uplift and subsequent weathering on the Cenozoic Os i record are likely small [51] , [52] . Carbon and osmium cycle modeling Enhanced volcanism and/or hydrothermal activity may represent the most parsimonious scenario to explain the modest negative Os i shift and atmospheric CO 2 rise during the MECO. However, a strong silicate weathering response to greenhouse warming through focused weathering of fresh basalts is in disagreement with the extensive carbonate dissolution observed in deep ocean basins [8] , [10] . Therefore, total continental weathering fluxes must have remained approximately constant during the event. Collectively, the available data indicate that CO 2 was added to the ocean-atmosphere system through enhanced volcanism, leading to warming, but was not neutralized through the silicate weathering feedback, leading to sustained ocean acidification. To test the plausibility of scenarios involving enhanced volcanism and/or diminished continental weathering during the MECO, we performed a series of carbon cycle simulations with the box model LOSCAR [23] by prescribing fluxes with the transient shift that is inferred from our Os i records (see Methods; Fig. 3 ; Supplementary Figs. 4 – 9 ). For consistency, we have also modeled the 187 Os/ 188 Os composition of the global ocean by applying the same LOSCAR carbon cycle fluxes as forcing to a box model of the Os cycle (see Methods; Supplementary Software 1). In addition to a ~0.05 decrease in the 187 Os/ 188 Os ratio of seawater, our target scenario for the MECO involves a rise in atmospheric CO 2 concentrations, a slight increase in the δ 13 C of dissolved inorganic carbon in the deep ocean, and a shoaling of the CCD over ~500 kyr [8] . Since there are no high-resolution p CO 2 records available for the MECO, the target scenario includes an approximate doubling of atmospheric CO 2 concentrations relative to middle Eocene background values of 500–1000 ppmv [11] , [53] . Furthermore, the magnitude of CCD change during the event possibly varied between the different ocean basins [10] , so we incorporate a conservative estimate of at least 500 m shoaling in the Atlantic and Pacific in our target scenario. Fig. 3 LOSCAR and Os cycle model simulations of the most likely MECO scenario. a Forcing for two scenarios involving a gradual, transient 20% increase in the volcanic CO 2 flux over ~500 kyr. The solid lines represent a scenario in which the silicate and carbonate weathering fluxes are allowed to vary in response to CO 2 forcing (normal weathering feedback), while the dashed lines represent a scenario in which these weathering fluxes are kept constant (diminished weathering feedback). Only the latter scenario corresponds to all observations. b Model response in the 187 Os/ 188 Os composition of the global ocean, shown against smoothed fits to the MECO Os i records from the study sites. c Model CCD response of different ocean basins, shown against carbonate content (wt%) records for different depths in the Atlantic, Indian and Pacific oceans as compiled by Sluijs et al [8] . d Model atmospheric p CO 2 response and pH response for the surface Atlantic and Pacific oceans. e Model δ 13 C response for the DIC of the deep Atlantic and Pacific oceans. For a full description of the LOSCAR model, see Zeebe [23] Full size image All model simulations result in a decrease in the 187 Os/ 188 Os ratio of seawater (Fig. 3 ; Supplementary Figs. 4 – 9 ). Although a gradual, linear increase in volcanism of 10–20% over ~500 kyr is sufficient to cause CO 2 accumulation in the ocean-atmosphere system, and hence global warming on MECO timescales, this scenario results in a deepening of the CCD instead of the observed shoaling (Fig. 3 ; Supplementary Fig. 4 ) [8] , [10] . A similar behavior of the CCD is observed in previous LOSCAR simulations of the MECO [8] and the Late Cretaceous warming episode [36] . Crucially, the model is only able to reproduce CO 2 rise in conjunction with shoaling of the CCD on these timescales if we invoke enhanced volcanism together with a diminished weathering feedback by maintaining the silicate and carbonate weathering fluxes constant (Fig. 3 ; Supplementary Fig. 5 ). Although the magnitude of this modeled CCD response is smaller than the shoaling inferred from deep-sea carbonate records [8] , [10] , we note that the model may underestimate CCD changes because it does not account for the additional effects of biological carbonate compensation [54] . Such a reduction in net carbonate production resulting from ocean acidification might amplify the CCD response for a given CO 2 rise. In all scenarios, the model reproduces the modest increase in deep-sea benthic foraminifer δ 13 C values during the event [9] , [10] because of a resulting decrease in carbonate versus constant organic carbon burial. Finally, the relatively rapid termination of the MECO is forced by a recovery of silicate weathering. We note that this does not need to represent a pronounced tectonic event, as the absolute magnitude of the flux imbalances is relatively small, but regionally enhanced weathering in the aftermath of the MECO would be consistent with observations from the Tethys region [55] . To reconcile our Os i records and model results with global warming and atmospheric CO 2 rise on MECO timescales [8] , [9] , [10] , [11] , we hypothesize that a long-term reduction in the strength of the negative silicate weathering feedback occurred in the Eocene [56] , [57] , due to a progressive reduction in the weatherability of the continents—the sum of all factors affecting chemical weathering other than climate [58] , [59] . For millions of years prior to the MECO, the Earth was generally characterized by high atmospheric CO 2 levels [53] and very warm climates [60] (Supplementary Fig. 10 ), as well as flat continental relief. Thick, cation-depleted soils developed and transport-limited weathering regimes prevailed [61] , [62] , and consequently the weatherability of Earth’s surface may have gradually decreased over the course of the Eocene. Indeed, such a progressive reduction in weathering feedback strength during the Eocene has been inferred from inverse modeling simulations of weathering fluxes based on Cenozoic p CO 2 and δ 13 C records [57] (Fig. 2c ). With the strength of the weathering feedback strongly diminished, a small increase in volcanism or hydrothermal activity would lead to the accumulation of large amounts of CO 2 in the ocean-atmosphere system, resulting in prolonged warming and ocean acidification during the MECO. Changes in weatherability have also been suggested to explain other episodes of apparent decoupling between silicate weathering and climate [59] , for example during major glaciations in the Paleozoic and Neoproterozoic [63] , [64] , [65] . Our interpretations of a limited weathering response during the MECO suggest that a variable silicate weathering feedback strength [57] can indeed act as a driver for sustained global warming on geological timescales, with potential importance to other enigmatic phases of carbon cycle change in Earth’s history. Moreover, a variable weathering feedback strength governed by the interplay between tectonics, climate and the weatherability of the continents fundamentally challenges the parameterization of the silicate weathering feedback in carbon cycle models, especially those used to model transient perturbations such as the OAEs and the PETM. We therefore argue that future studies of these events should focus on exploring changes in temperature, atmospheric CO 2, and the CCD in conjunction with the strength of the weathering feedback. Sampling The samples used in this study were derived from middle Eocene sedimentary units from three different sites: organic-rich sediments from ODP Site 959 in the equatorial Atlantic along the African continental margin, carbonate-rich pelagic sediments from ODP Site 1263 on the Walvis Ridge in the south Atlantic, and carbonate-rich pelagic sediments from IODP Site U1333 in the equatorial Pacific (Supplementary Fig. 1 ). The total organic carbon (TOC) contents of these middle Eocene sediments range between 0.1 and 2%, with the highest TOC abundances occurring at Site 959 [66] . Rock samples of 20–40 g were selected across the middle Eocene interval between approximately 42 and 38 Ma, with the highest sampling resolution across the MECO. Analyses Bulk samples were freeze-dried or oven-dried at 50 °C and subsequently powdered using a ceramic pestle and mortar, in order to homogenize the Re and Os within the samples. Contact with metal surfaces was avoided so as not to contaminate the sample set. All Re and Os isotope analyses were performed at the Laboratory for Source Rock and Sulfide Geochronology and Geochemistry, and the Arthur Holmes Laboratory at the Durham Geochemistry Centre, Durham University (UK). Samples were digested in a CrO 3 -H 2 SO 4 solution (0.25 g/g CrO 3 in 8 mL of 4 N H 2 SO 4 ) following the well-established methods of Selby & Creaser [67] , which have been shown to significantly limit the contribution of detrital Re and Os to the hydrogenous fraction bound to organic matter. Powdered samples of approximately 0.3–1 g were loaded into Carius tubes with a known amount of 185 Re + 190 Os tracer solution (spike) and dissolved in 8 mL of CrO 3 -H 2 SO 4 solution. The Carius tubes were then sealed and heated in an oven at 220 °C for 48 h. Osmium was isolated from the CrO 3 -H 2 SO 4 sample solution by using solvent extraction with chloroform (CHCl 3 ), and then back extracted by hydrobromic acid (HBr). The Os was further purified through micro distillation. Rhenium was isolated by evaporating 1 mL of the CrO 3 –H 2 SO 4 sample solution to dryness, followed by solvent extraction involving sodium hydroxide (NaOH) and acetone (C 3 H 6 O) [68] , [69] . The Re was further purified by anion chromatography. Following purification, the Re and Os fractions were loaded onto Ni and Pt filaments, respectively, together with 0.5 μL BaNO 3 and BaOH activator solutions, respectively [67] . Rhenium and osmium isotope ratios were determined by negative thermal ionization mass spectrometry, using Faraday cups for Re and a Secondary Electron Multiplier for Os in peak-hopping mode. Re and Os isotope ratios were corrected for instrumental mass fractionation, as well as spike and blank contributions. Procedural blanks for Re and Os in this study were 12 ± 3 pg/g and 0.07 ± 0.05 fg/g, respectively, with an 187 Os/ 188 Os value of 0.25 ± 0.15 ( n = 3). The 187 Re/ 188 Os and 187 Os/ 188 Os uncertainties (2σ) include full propagation of uncertainties in weighing, mass spectrometer measurements, spike calibrations, blank corrections, and reproducibility of standards. The 187 Os/ 188 Os initial ratios (Os i ) were calculated by correcting for post-depositional 187 Re decay over time with the following equation: 
    ^187Os/^188Os_initial( Os_i) = ^187Os/^188Os_measured - ^187Re/^188Os_measured∗( e^λ t - 1)
 (1) where λ is the 187 Re decay constant (1.666 · 10 −11 yr −1 ) [70] and t is the age of the rock. Given the high Re abundances in the organic-rich sediments from Site 959, we have used best estimates for the depositional ages of each of these samples. An age of 40 Ma was used for all samples from Sites 1263 and U1333, because improved age estimates would result in variations in Os i values of 0.1% or less on average. All results are listed in Supplementary Data 1 . The Re–Os isotopic system is expected to have remained closed for the sample set, given that the cores were all fresh, unweathered, and showed no evidence of post-depositional events (e.g., veining, etc.). Further, where the Re–Os data has sufficient spread in isochron plot space to yield statistically robust isochrons, a geologically reasonable Re–Os isochron age is obtained (e.g., Site 959; see below for details). Evaluation of Re and Os data Although the studied samples were collected for evaluating changes in Os i rather than establishing isochrons, the Re–Os data of the sediments from Site 959 show a positive correlation between 187 Re/ 187 Os and 187 Os/ 188 Os, which results in an isochron age that is in good agreement with the age of the MECO between 40.5 and 40.0 Ma (Supplementary Figs. 2 , 3 ). In contrast, the 187 Re/ 187 Os and 187 Os/ 188 Os data for Sites 1263 and U1333 do not have sufficient spread in isochron plot space, and hence cannot yield statistically geologically meaningful age estimates. Age models We adopt the age model of Cramwinckel et al. [13] for Site 959 (Supplementary Fig. 11 ). This is based on initial [71] and recently improved [13] calcareous nannofossil biostratigraphy. The model also uses the long-term 187 Os/ 188 Os minimum at 34.65 Ma recorded at this site [26] , and TEX 86 data that mark the MECO warming [13] . Moreover, we use the highest TEX 86 value during the MECO peak warming and the lowest TEX 86 value at the onset of the MECO as reported by Cramwinckel et al. [13] to tentatively correlate to minima and maxima in the δ 18 O records of Bohaty et al. [10] , which were assigned ages of 40.06 and 40.52 Ma, respectively. Better age models are available for the other two sites. For Site 1263, we use a published age model [10] based on magnetostratigraphy and bulk carbonate δ 18 O and δ 13 C chemostratigraphy. For Site U1333, an astronomically calibrated magnetostratigraphic age model [72] was used in combination with calcareous nannofossil events [73] . 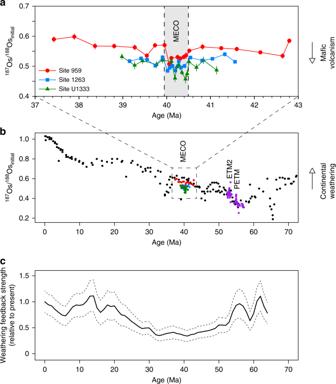Fig. 2 Comparison of Osirecords from the MECO with Osirecords from the PETM and ETM2, shown against the overall Osievolution of the Cenozoic and the relative weathering feedback strength of the Cenozoic.aMECO data from Site 959 (in red), Site 1263 (in blue) and Site U1333 (in green) plotted against age (GTS2012)74. See Methods for discussion of the age models for the study sites.bMECO data from Sites 959, 1263, and U1333 (this study); PETM and ETM2 data from DSDP Site 549 (in purple) as published in Peucker-Ehrenbrink & Ravizza15; Cenozoic data from ferromanganese crusts D11 and CD29 (in black) as published in Klemm et al.27and Burton28, respectively, based on the updated age model of Nielsen et al.29.cModel estimates of the relative continental weathering feedback strength of the Cenozoic as published in Caves et al.57, based on their CO2scenario 1 and a logarithmic expression for the weathering feedback 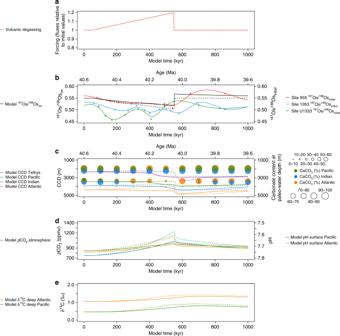Fig. 3 LOSCAR and Os cycle model simulations of the most likely MECO scenario.aForcing for two scenarios involving a gradual, transient 20% increase in the volcanic CO2flux over ~500 kyr. The solid lines represent a scenario in which the silicate and carbonate weathering fluxes are allowed to vary in response to CO2forcing (normal weathering feedback), while the dashed lines represent a scenario in which these weathering fluxes are kept constant (diminished weathering feedback). Only the latter scenario corresponds to all observations.bModel response in the187Os/188Os composition of the global ocean, shown against smoothed fits to the MECO Osirecords from the study sites.cModel CCD response of different ocean basins, shown against carbonate content (wt%) records for different depths in the Atlantic, Indian and Pacific oceans as compiled by Sluijs et al8.dModel atmosphericpCO2response and pH response for the surface Atlantic and Pacific oceans.eModel δ13C response for the DIC of the deep Atlantic and Pacific oceans. For a full description of the LOSCAR model, see Zeebe23 All ages were adjusted to the framework of the GTS 2012 [74] and tie points for the age models are listed in Supplementary Tables 1 , 2 and 3 . Calculating changes in Os fluxes across the MECO The 187 Os/ 188 Os composition of seawater is controlled by the balance between input fluxes from continental, mantle-derived, and extraterrestrial sources. However, the flux of extraterrestrial Os is generally assumed to be negligible and constant [75] , [76] , so our Os i records can be used to directly infer changes in relative contributions of the continental and mantle-derived Os sources across the MECO. To evaluate an increase in the mantle-derived Os flux, we developed a progressive, two-component mixing model for the release of Os from mantle-derived basalts that incorporates both the Os abundance and 187 Os/ 188 Os composition of seawater and basalts. This model is an adaptation of the two-component mixing model for strontium (Sr) isotopes of Faure (1986, Equations (9.2) and (9.10)) [77] , with modifications to consider the larger range of Os isotope variations in comparison to Sr isotope variations. From the relative molar concentrations of natural Os isotopes, we know: 
    [ Os] - [  ^187Os]/[  ^188Os] = 7.4
 (2) where [Os] represents the molar concentration (in mol/kg) of total Os (i.e., 186 Os + 187 Os + 188 Os + 189 Os + 190 Os + 192 Os), and [ 187 Os] and [ 188 Os] represent the molar concentrations (in mol/kg) of 187 Os and 188 Os, respectively [78] . Equation ( 2 ) can be rewritten as: 
    [  ^187Os] = R/7.4 + R[ Os]
 (3) 
    [  ^188Os] = 1/7.4 + R[ Os]
 (4) where R = [ 187 Os]/[ 188 Os]. Two-component mixing between seawater and basalts can then be expressed for both 187 Os and 188 Os as: 
    [  ^187Os]_mix = [  ^187Os]_sw∗ M_sw + [  ^187Os]_bas∗ M_bas/M_sw + M_bas
 (5) 
    [  ^188Os]_mix = [  ^188Os]_sw∗ M_sw + [  ^188Os]_bas∗ M_bas/M_sw + M_bas
 (6) where M represents the mass of a component (in kg) and the subscripts sw, bas and mix represent seawater, basalts and the eventual mix between the two, respectively. We now define: 
    Δ M_bas = M_bas/M_sw,initial
 (7) 
    f = Δ M_bas/M_sw,progressive + Δ M_bas = Δ M_bas/M_mix
 (8) where Δ M bas is an infinitesimal representing the mass of basalts added during a mixing step relative to the mass of seawater initially present, and f represents the amount of basalts added during a mixing step relative to the total amount of seawater and basalts present during progressive mixing ( M mix ). Equations ( 3 )–( 8 ) can then be combined as follows: 
    [            [  ^187Os]_mix = f ∗[  ^187Os]_bas + ( 1 - f) ∗[  ^187Os]_sw; 70pt= f ∗R_bas/7.4 + R_bas[ Os]_bas + ( 1 - f) ∗R_sw/7.4 + R_sw[ Os]_sw ]
 (9) 
    [     [  ^188Os]_mix = f ∗[  ^188Os]_bas + ( 1 - f) ∗[  ^188Os]_sw; 70pt= f ∗1/7.4 + R_bas[ Os]_bas + ( 1 - f) ∗1/7.4 + R_sw[ Os]_sw ]
 (10) Finally, dividing equation ( 9 ) by equation ( 10 ) yields: 
    [ R_mix = [  ^187Os]_mix/[  ^188Os]_mix = f ∗R_bas/7.4 + R_bas[ Os]_bas + ( 1 - f) ∗R_sw/7.4 + R_sw[ Os]_sw/f ∗1/7.4 + R_bas[ Os]_bas + ( 1 - f) ∗1/7.4 + R_sw[ Os]_sw ]
 (11) where R is the 187 Os/ 188 Os composition of the corresponding components (i.e., seawater, basalts, and the eventual mix between the two). Equations ( 7 )–( 11 ) can then be used to estimate the extent of mixing between seawater and basalts during the MECO by progressively calculating R mix until our observed Os i shift is reproduced (see Supplementary Data 2 ). We assumed the pre-MECO 187 Os/ 188 Os ratio of seawater to be ~0.55 based on an average of pre-MECO Os i values recorded for the three sites and the Os concentration of seawater to be 10 ppq (~53 fmol/kg, similar to present-day values) [14] . Furthermore, we used an 187 Os/ 188 Os ratio of 0.13 for the mantle and mantle-derived basalts [79] , [80] , as well as an Os abundance of 1 ppt (~5.3 pmol/kg) for basalts [80] . Finally, we assumed that the maximum amount of basalt that can theoretically be added to seawater represents ~1% of the total mass of the ocean, as estimated for OAE2 [31] , [81] , and used increments of 0.01% for the value of Δ M bas . Based on an Os i shift of 0.05 from the pre-MECO value of ~0.55 to a peak MECO value of ~0.50, we calculated a relative increase in the mantle-derived Os flux of ~13% across the event, which would equal the addition of Os from basalts with a mass of ~0.13% relative to the total mass of the ocean (Supplementary Data 2 ). Similar results are obtained if we estimate the relative increase in the 188 Os flux, rather than the total Os flux. It is important to note that mantle-derived Os could also have been released to seawater through direct addition from magmatic degassing or hydrothermal inputs instead of basalt dissolution, but regardless of the mechanism, a ~13% increase in the mantle-derived Os flux during the MECO would be sufficient to reproduce our observed Os i shift and would correspond to the cumulative release of ~9.4 · 10 6 mol of mantle-derived Os. We also performed our calculations with the Os i values of each individual site: for Site 959, an Os i shift from 0.560 to 0.505 would yield a relative increase in the mantle-derived Os flux of ~14%; for Site 1263, an Os i shift from 0.530 to 0.485 would yield an increase of ~12%; for Site U1333, an Os i shift from 0.515 to 0.460 would yield an increase of ~16%. These differences are most likely to be attributed to the resolution of our records. To accommodate for this range of flux estimates, we adopted a best estimate of 10–15% for the increase in the mantle-derived Os flux during the MECO, but also explored the effects of an increase of up to 20% because we are unlikely to have sampled the lowest Os i values in any of our records due to the relatively low resolution of our dataset. LOSCAR and Os cycle modeling Carbon cycle simulations were performed using the Long-term Ocean-atmosphere-Sediment CArbon cycle Reservoir (LOSCAR) model [23] . In this box model, modified from Walker and Kasting [82] , carbon and several other biogeochemical tracers (e.g., alkalinity, phosphate, oxygen) are cycled through atmospheric and oceanic reservoirs. The model ocean is coupled to a sediment module and consists of surface-water, intermediate-water, and deep-water boxes of the four main Paleogene ocean basins (Atlantic, Indian, Pacific and Tethys). The model is designed to simulate the PETM at 56 Ma, but the minor changes in paleogeography compared to the middle Eocene at 40 Ma are not of relevance to the simple LOSCAR model. In these simulations, we use default parameter settings for the Paleogene setup. Equilibrium p CO 2 is set at 750 ppm, consistent with p CO 2 estimates based on planktic foraminifer boron isotope ratios (δ 11 B) [53] , and by default, silicate and carbonate weathering are implemented in the model as a feedback response to atmospheric CO 2 concentrations. The CCD definition follows the default LOSCAR setup and is taken as the sediment depth level at which sedimentary CaCO 3 contents fall below 10 wt%. We explored the effects of changes in volcanism and/or continental weathering with the constraints from our Os i records to assess which scenario is able to reproduce a more realistic MECO target. We first simulated several scenarios with a gradual, linear increase in the volcanic CO 2 flux (+10, +15, and +20%) over ~500 kyr, either while allowing the silicate and carbonate weathering fluxes to vary in response to CO 2 forcing (Supplementary Fig. 4 ), or while maintaining these weathering fluxes at constant values (Supplementary Fig. 5 ). Subsequently, we performed several simulations invoking silicate weathering as a forcing rather than a feedback, by prescribing a gradual, linear decrease in the silicate weathering flux (−10, −15, and −20%) over ~500 kyr, while keeping the volcanic CO 2 flux and the carbonate weathering flux at constant values (Supplementary Fig. 6 ). Finally, we tested the effect of an increase in volcanism (+5%) combined with a decrease in silicate weathering (−5%) (Supplementary Fig. 7 ); the effect of a combined decrease in silicate and carbonate weathering (both −10%) (Supplementary Fig. 8 ); and the effect of a decrease in silicate weathering (−10%) while maintaining a carbonate weathering feedback (Supplementary Fig. 9 ). For an overview of all model scenarios, see Supplementary Table 4 . In order to demonstrate that our LOSCAR model simulations are consistent with the Os i records, the scenarios outlined above were also applied to a separate box model of the Os cycle. This Os cycle model is inspired by the work of Richter & Turekian [83] and many subsequent studies, including Peucker-Ehrenbrink & Ravizza [14] . We fully derive the equations used to model the Os cycle in the ocean below. We first define N as the total molar inventory of Os (including all Os isotopes) in seawater, and 187 N and 188 N as the molar inventories of 187 Os and 188 Os in seawater, respectively. The 187 Os/ 188 Os composition of seawater ( R sw ) is thus expressed as: 
    R_sw =  ^187N/ ^188N
 (12) Subsequently, changes in R sw over time can be written as: 
    [ dR_sw/dt = d/dt(  ^187N/ ^188N) =  ^188Nd^187N/dt -  ^187Nd^188N/dt/(  ^188N)^2 = 1/ ^188N[ d^187N/dt - R_swd^188N/dt] ]
 (13) Multiplying equation ( 13 ) by 188 N gives: 
    ^188NdR_sw/dt = d^187N/dt - R_swd^188N/dt
 (14) Changes in N , 187 N and 188 N over time can then be written as follows: 
    dN/dt = F_riv + F_hyd + F_ext - F_sed
 (15) 
    [ d^187N/dt = F_riv( [  ^187Os]/[ Os])_riv +  F_hyd( [  ^187Os]/[ Os])_hyd+  F_ext( [  ^187Os]/[ Os])_ext -  F_sed( [  ^187Os]/[ Os])_sed ]
 (16) 
    [ d^188N/dt = F_riv( [  ^188Os]/[ Os])_riv +  F_hyd( [  ^188Os]/[ Os])_hyd +  F_ext( [  ^188Os]/[ Os])_ext -  F_sed( [  ^188Os]/[ Os])_sed ]
 (17) where F represents the fluxes of Os (in mol/yr) from and to various reservoirs and the subscripts sw, riv, hyd, ext and sed represent seawater, riverine, hydrothermal, extraterrestrial and sediment reservoirs, respectively [14] , [83] . Substituting equations ( 3 ) and ( 4 ) into equations ( 16 ) and ( 17 ), respectively, yields: 
    [ d^187N/dt = F_rivR_riv/7.4 + R_riv + F_hydR_hyd/7.4 + R_hyd+  F_extR_ext/7.4 + R_ext - F_sedR_sed/7.4 + R_sed ]
 (18) 
    [ d^188N/dt = F_riv1/7.4 + R_riv + F_hyd1/7.4 + R_hyd+ F_ext1/7.4 + R_ext - F_sed1/7.4 + R_sed ]
 (19) Finally, substituting equations ( 18 ) and ( 19 ) into equation ( 14 ) and combining with equation ( 4 ) results in: 
    [ N/7.4 + R_swdR_sw/dt = F_rivR_riv - R_sw/7.4 + R_riv + F_hydR_hyd - R_sw/7.4 + R_hyd+ F_extR_ext - R_sw/7.4 + R_ext - F_sedR_sed - R_sw/7.4 + R_sed ]
 (20) which relates changes in R sw over time to the fluxes of total Os ( F ), the 187 Os/ 188 Os compositions of these fluxes ( R ) and the amount of total Os in the ocean ( N ). Because there is no isotopic fractionation associated with Os burial (i.e., R sed = R sw ), the net effect of the sedimentary Os flux ( F sed ) in equation ( 20 ) is zero. Together, equations ( 15 ) and ( 20 ) can be used to simulate any transient perturbation of the Os cycle. We first constructed a steady state model based on flux estimates and 187 Os/ 188 Os values for the present-day Os cycle with a 187 Os/ 188 Os ratio of seawater of 1.06 (see Supplementary Table 5 ). For the middle Eocene Os cycle, we assumed that the total Os inventory and the total input and output fluxes of Os are similar to present-day values, and recalculated the steady state riverine and hydrothermal Os fluxes for the pre-MECO 187 Os/ 188 Os ratio of seawater of 0.55 by assuming that the 187 Os/ 188 Os composition of these fluxes has remained unchanged. Subsequently, we used scaled silicate weathering and volcanic degassing fluxes from the LOSCAR model simulations to force our model of the Os cycle. The modeled changes in the 187 Os/ 188 Os ratio of seawater are included in the respective figures of all model scenarios (Fig. 3 of the main text and Supplementary Figs. 4 – 9 ). The full code used to perform the Os cycle model simulations is included as an R script in Supplementary Software 1. Data availability The authors declare that all data supporting the results of this study are available in the Supplementary Information files associated with this manuscript.